Occupancy of tissue-specificcis-regulatory modules by Otx2 and TLE/Groucho for embryonic head specification Head specification by the head-selector gene, orthodenticle ( otx ), is highly conserved among bilaterian lineages. However, the molecular mechanisms by which Otx and other transcription factors (TFs) interact with the genome to direct head formation are largely unknown. Here we employ ChIP-seq and RNA-seq approaches in Xenopus tropicalis gastrulae and find that occupancy of the corepressor, TLE/Groucho, is a better indicator of tissue-specific cis -regulatory modules (CRMs) than the coactivator p300, during early embryonic stages. On the basis of TLE binding and comprehensive CRM profiling, we define two distinct types of Otx2- and TLE-occupied CRMs. Using these devices, Otx2 and other head organizer TFs (for example, Lim1/Lhx1 (activator) or Goosecoid (repressor)) are able to upregulate or downregulate a large battery of target genes in the head organizer. An underlying principle is that Otx marks target genes for head specification to be regulated positively or negatively by partner TFs through specific types of CRMs. The bilaterian head forms in the most anterior part of the developing embryo. In early embryogenesis, the head-selector, Otx (orthodenticle), a homeodomain-containing transcription factor (TF), is expressed in the head region. In contrast, homeotic selector Hox cluster TFs are expressed along the anteroposterior axis of the trunk and tail [1] , [2] . Otx homeodomain proteins are conserved among bilaterians, from flies to humans, and their functions are essential for proper head formation [2] . However, little is known about the mechanisms by which Otx proteins confer different head structures among different species, or about the types of cis -regulatory modules (CRMs) utilized by Otx proteins. To resolve these questions, we carried out comprehensive analyses of Otx target genes and characterized their CRMs, using thousands of synchronized whole Xenopus gastrula embryos. In developmental biology, an organizer refers to a group of cells or a small piece of tissue that induces surrounding cells to develop into specific tissues or organs. During amphibian embryogenesis, the gastrula organizer known as the Spemann–Mangold organizer initiates gastrulation movements and establishes the basic body plan. The organizer consists of two different regions—head and trunk organizers, which effect anteroposterior patterning of the neuroectoderm [3] . Genes for homeodomain proteins, Otx2, Lim1 (=Lhx1) and Goosecoid (Gsc), are expressed in the head organizer to specify head structures [4] , [5] , [6] , [7] , [8] , [9] . The transcriptional regulatory networks underlying the Xenopus organizer have been studied extensively, especially focusing on regulation of gsc [10] . Previous work has shown that Otx2 and Lim1 upregulate head organizer genes such as gsc and cerberus , and that Gsc downregulates trunk genes such as brachyury and wnt8a [10] , [11] , [12] , [13] , [14] , [15] , [16] . At present, the regulatory principle governing Otx2, Lim1 and Gsc remains unsolved. Using X. tropicalis gastrula embryos, we carry out genome-wide chromatin immunoprecipitation sequencing (ChIP-seq) analysis for Otx2, Lim1, Gsc, the general coactivator, p300, the general corepressor, TLE/Groucho, and histone marks. In addition, RNA sequencing (RNA-seq) analysis is performed on embryos knocking down these TFs, as well as dissected embryonic tissue fragments. Our analyses reveal for the first time that TLE occupancy around the CRM is a better indicator of tissue-specific CRM activity than is p300 occupancy. On the basis of molecular interaction studies among Otx2, Lim1 and Gsc via specific CRMs, we propose a regulatory model, in which Otx2 binding on the genome represents marking of head-induction processes in early vertebrate gastrula embryos by simultaneously upregulating a large battery of target genes in cooperation with Lim1, and downregulating others in concert with Gsc ( Supplementary Fig. 1 ). The simplicity of this mode of head specification may explain the evolutionarily conservation of the head-selector Otx. Cooperation of head organizer TFs in head formation Previous studies in mice deficient in Otx2, Lim1 and Gsc have shown that head formation can proceed without Gsc, but not without Otx2 and Lim1 [17] , [18] , [19] , [20] , [21] . Because lim1 , gsc , otx2 and its paralog, otx5 , are co-expressed in the organizer of X. tropicalis early gastrulae similar to X. laevis [16] , [22] , [23] ( Fig. 1a ), in X. tropicalis we knocked down combinations of Otx2, Otx5, Lim1 and Gsc using antisense morpholino oligos (MOs; Fig. 1b ; see Supplementary Fig. 2 for MO specificity). Morphants injected with lim1/otx2/otx5 or otx2/otx5/gsc triple MOs or all four MOs exhibited more severe head-reduced phenotypes than single or double morphants ( Supplementary Fig. 2C ). Sagittal sections and brain marker gene expression confirmed that anterior structures such as the forebrain, midbrain and foregut were shrunk in the morphants ( Fig. 1b ). Compared with other single morphants, otx2 morphants exhibited more severe head defects, in which about 25% of embryos had small heads with trace eyes. This may be at least partly due to otx2 ’s expression in the anterior neural tissue and later in the brain, in addition to the head organizer [8] , [9] . gsc single morphants exhibited cyclopic phenotypes ( Supplementary Fig. 2C ), similar to those reported in X. laevis [24] . In mice, Lim1 - or Otx2 -deficient embryos display a total lack of head structures, much more severe defects than seen in lim1 or otx2 single morphants in X. tropicalis . Less serious defects in Xenopus may be due to incomplete knockdown by MOs. Nevertheless, knockdown data indicate that Otx2, Otx5, Lim1 and Gsc all contribute to head formation cooperatively, but each works in a different way. 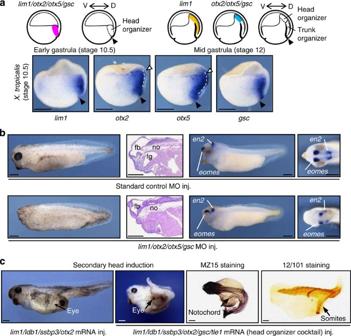Figure 1: Phenotypes of loss- and gain-of-function of head organizer TFs in frogs. (a) Expression patterns ofotx2, otx5, lim1andgscinXenopusgastrula embryos. Schematic representation shows co-expression oflim1,otx2,otx5andgscin the head organizer4,5,6,7,8,9,16,22,23,56andlim1expression in the trunk organizers16,56. A double-headed arrow indicates the dorsal (D) and ventral (V) axis. Co-expression of these genes inX. tropicalisearly gastrula embryos was shown within situhybridization using hemisections. In anterior neuroectoderm,otx2is weakly expressed, whileotx5is more strongly expressed. Arrowhead, dorsal blastopore; open arrowhead, expression in the anterior neuroectoderm; and dashed line, boundary of ectoderm and mesoderm. (b) Loss-of-function analysis inX. tropicalis. Phenotypes of normal embryos (control morphants) and head-reduced embryos (lim1/otx2/otx5/gscmorphants) are shown. Sagittal section and whole mountin situhybridization of the telencephalon marker (eomes) and the midbrain–hindbrain boundary marker (en2) showed that forebrain, midbrain and foregut were shrunk in head-reduced embryos. Note that the notochord reached the anterior-most region in the morphant. Tailbud embryos are shown in lateral (anterior to the left; three left panels) or dorsoanterior (right-most panels) views. fb, forebrain; fg, foregut; no, notochord. (c) Gain-of-function analysis inX. laevis. Left panels show lateral views of a secondary head with one eye generated after ventral injection (inj.) of a cocktail of mRNAs as indicated. Right panels show immunostaining of head organizer cocktail-injected embryos against notochord by MZ15 (dorsal view of the same embryo as shown in the left panel) and somites by 12/101 (lateral view), respectively. Scale bar, 250 μm. Figure 1: Phenotypes of loss- and gain-of-function of head organizer TFs in frogs. ( a ) Expression patterns of otx2, otx5, lim1 and gsc in Xenopus gastrula embryos. Schematic representation shows co-expression of lim1 , otx2 , otx5 and gsc in the head organizer [4] , [5] , [6] , [7] , [8] , [9] , [16] , [22] , [23] , [56] and lim1 expression in the trunk organizers [16] , [56] . A double-headed arrow indicates the dorsal (D) and ventral (V) axis. Co-expression of these genes in X. tropicalis early gastrula embryos was shown with in situ hybridization using hemisections. In anterior neuroectoderm, otx2 is weakly expressed, while otx5 is more strongly expressed. Arrowhead, dorsal blastopore; open arrowhead, expression in the anterior neuroectoderm; and dashed line, boundary of ectoderm and mesoderm. ( b ) Loss-of-function analysis in X. tropicalis . Phenotypes of normal embryos (control morphants) and head-reduced embryos ( lim1/otx2/otx5/gsc morphants) are shown. Sagittal section and whole mount in situ hybridization of the telencephalon marker ( eomes ) and the midbrain–hindbrain boundary marker ( en2 ) showed that forebrain, midbrain and foregut were shrunk in head-reduced embryos. Note that the notochord reached the anterior-most region in the morphant. Tailbud embryos are shown in lateral (anterior to the left; three left panels) or dorsoanterior (right-most panels) views. fb, forebrain; fg, foregut; no, notochord. ( c ) Gain-of-function analysis in X. laevis . Left panels show lateral views of a secondary head with one eye generated after ventral injection (inj.) of a cocktail of mRNAs as indicated. Right panels show immunostaining of head organizer cocktail-injected embryos against notochord by MZ15 (dorsal view of the same embryo as shown in the left panel) and somites by 12/101 (lateral view), respectively. Scale bar, 250 μm. Full size image In gain-of-function experiments, we injected combinations of mRNAs encoding Lim1, Ldb1, Ssbp3, Otx2, Gsc and Tle1 into the ventral equatorial region ( Fig. 1c ). Ldb1 and Ssbp3 are Lim1 cofactors that activate Lim1 [25] , [26] . Tle1 is an Otx2- and Gsc-binding corepressor [27] , [28] . Lim1/Ldb1/Ssbp3 together with Otx2, Gsc/Tle1 or both induce secondary head structures that were never observed after overexpression of Lim1/Ldb1/Ssbp3 or Otx2/Gsc/Tle1 ( Supplementary Fig. 3A ). Furthermore, the combination of Lim1, Ldb1, Ssbp3, Otx2, Gsc and Tle1 showed significantly higher rates of secondary head induction than other combinations ( Supplementary Fig. 3A ). Therefore, we refer to it as the ‘head organizer cocktail.’ This is the first demonstration that Lim1, Otx2 and Gsc synergistically generate secondary head structures in vertebrate embryos. As demonstrated by immunostaining, the secondary axis induced by the head organizer cocktail contained the notochord and somites ( Fig. 1c ). This kind of phenotype is usually called a complete axis, but unlike a Wnt-induced axis, the secondary axis resulting from the head organizer cocktail exhibited a shortened trunk accompanied by a bent tail and an open blastopore ( Fig. 1c ). The animal cap assay demonstrated that the head organizer cocktail induced head organizer genes ( chordin , gsc and cerberus ), but not the trunk organizer gene ( brachyury ) and the muscle marker gene ( actc1 ; Supplementary Fig. 3B ). Thus, the head organizer cocktail induces primarily the head and secondarily the trunk, possibly due to both anteriorizing and dorsalizing activities of this cocktail. Features of head organizer TF-occupied CRMs To identify CRMs and in vivo target genes for Otx2, Lim1 and Gsc in the organizer, we performed ChIP-seq using X. tropicalis early gastrula embryos. At this stage of embryonic development, these three genes are strongly co-expressed in the head organizer region ( Fig. 1a ). Because cross-reactivity of our anti-Otx2 antibody to Otx5 protein is limited [16] , and because otx2 expression in anterior neuroectoderm just began at this stage ( Fig. 1a ), the ChIP-seq data of Otx2 was regarded as coming mainly from the head organizer. To uncover potential enhancer and silencer functions of CRMs and their epigenetic states, we also performed ChIP-seq for p300, TLE, monomethylated histone H3 lysine 4 (H3K4me1) and acetylated histone H3 lysine 27 (H3K27ac). In addition, we utilized previously reported ChIP-seq data for trimethylated histone H3 lysine 27 (H3K27me3) and RNA polymerase II (RNAP2) [29] . ChIP-seq peak data were validated using quantitative PCR (qPCR; Supplementary Fig. 4A–E ), another peak-calling algorithm ( Supplementary Tables 1 and 2 ; see Methods for details) and the following specific and overall peak analyses: (i) ChIP-seq peaks of all TFs were detected at a well-studied CRM, gsc -U1 (refs 10 , 11 , 16 ) ( Fig. 2a ); (ii) motif discovery analysis for Otx2, Lim1 or Gsc ChIP-seq peaks showed strong enrichment of their known binding motifs [11] , [12] , [16] , [30] , [31] ( Fig. 2b ; see Supplementary Fig. 5 for details); (iii) p300 peaks were correlated well with enhancer histone modifications, H3K4me1 and H3K27ac, but not with the repressive histone mark H3K27me3, as expected ( Fig. 2c ); (iv) average peak profiles around transcription start sites (TSSs) showed that Otx2, Lim1, p300, H3K4me1 and H3K27ac, but not Gsc and TLE, were strongly enriched at TSS ( Fig. 2d ), implying that transcriptional activators and coactivators (Otx2, Lim1 and p300), but not repressors and corepressors (Gsc and TLE), preferably associate with TSS; (v) Pearson correlation coefficient analysis using ChIP-seq enrichment data in 200 base pair (bp) windows across the entire genome ( Fig. 2e ) showed that Lim1 was correlated with p300 ( R =0.328) more strongly than with TLE ( R =0.202), whereas Otx2 was correlated with TLE ( R =0.572) more strongly than with p300 ( R =0.473). In this matrix, Gsc was correlated with TLE ( R =0.183) more strongly than with p300 ( R =0.170), but only marginally; (vi) when co-occupancies of ChIP-seq peaks (overlaps of peaks) were compared, correlation between Gsc and TLE became much more prominent (15.9 versus 6.6% in the line of Gsc in Fig. 2f ) than that in the correlation matrix. Results of (iv–vi) are consistent with previous reports that Gsc and Lim1 function exclusively as a repressor and an activator, respectively, while Otx2 has both functions [11] , [12] , [27] , [28] , [32] , [33] . These analyses validated the quality of our ChIP-seq data. 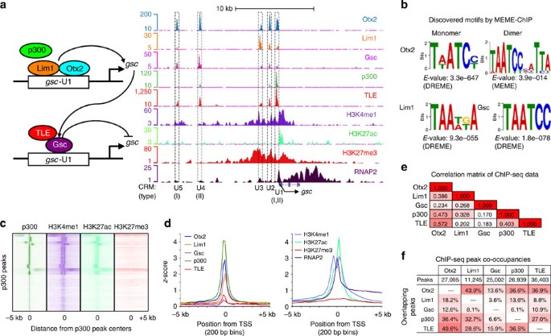Figure 2: Validations of ChIP-seq data. (a) ChIP-seq data surrounding a well-known target gene,gsc. Transcriptional regulatory model ofgscgene throughgsc-U1 is shown on the left. Lim1 and Otx2 activategscand Gsc represses itself viagsc-U111,16. In the genome browser representation, the ordinate shows enrichment against input control DNA for five TFs, or sequence tag enrichment for epigenetic marks, as indicated. Refseq gene models are shown with TSSs (bent arrows). According to the relative location of CRMs with respect to TSSs, the CRM was named as U-CRM (upstream CRM) or D-CRM (downstream CRM) and indicated by dashed boxes. Type I and type II CRMs (see text for definitions) are indicated in parentheses. (b) Enriched sequence motifs in Otx2, Lim1 and Gsc ChIP-seq peaks. Using the MEME-ChIP program, known binding motifs were found as enriched motifs. For Otx2, both monomer- and dimer-binding motifs were found.E-values were shown with the algorithm. (c) Clustered heatmap representations of ChIP-seq data around p300 peaks. Each genomic position was clustered according to p300 ChIP-seq data (k=10). H3K4me1 and H3K27ac, but not H3K27me3 data, were correlated with p300 peaks. (d) DNA occupancies of TFs (left) and epigenetic marks (right) around TSS. AverageZ-scores of ChIP-seq signals were plotted. (e) A matrix of Pearson correlation coefficients of ChIP-seq enrichment between each pair of TFs. (f) A table of proportions of ChIP-seq peak overlaps between each pair of TFs. Figure 2: Validations of ChIP-seq data. ( a ) ChIP-seq data surrounding a well-known target gene, gsc . Transcriptional regulatory model of gsc gene through gsc -U1 is shown on the left. Lim1 and Otx2 activate gsc and Gsc represses itself via gsc -U1 [11] , [16] . In the genome browser representation, the ordinate shows enrichment against input control DNA for five TFs, or sequence tag enrichment for epigenetic marks, as indicated. Refseq gene models are shown with TSSs (bent arrows). According to the relative location of CRMs with respect to TSSs, the CRM was named as U-CRM (upstream CRM) or D-CRM (downstream CRM) and indicated by dashed boxes. Type I and type II CRMs (see text for definitions) are indicated in parentheses. ( b ) Enriched sequence motifs in Otx2, Lim1 and Gsc ChIP-seq peaks. Using the MEME-ChIP program, known binding motifs were found as enriched motifs. For Otx2, both monomer- and dimer-binding motifs were found. E -values were shown with the algorithm. ( c ) Clustered heatmap representations of ChIP-seq data around p300 peaks. Each genomic position was clustered according to p300 ChIP-seq data ( k =10). H3K4me1 and H3K27ac, but not H3K27me3 data, were correlated with p300 peaks. ( d ) DNA occupancies of TFs (left) and epigenetic marks (right) around TSS. Average Z -scores of ChIP-seq signals were plotted. ( e ) A matrix of Pearson correlation coefficients of ChIP-seq enrichment between each pair of TFs. ( f ) A table of proportions of ChIP-seq peak overlaps between each pair of TFs. Full size image Because short genomic regions targeted by multiple TFs are proposed to function as CRMs in mouse embryonic stem cells [34] , we define CRMs as overlapping binding regions for two or more of the five factors, Otx2, Lim1, Gsc, p300 and TLE ( Table 1 ). Overlapping means that two peaks share more than 120 bases (see Methods for details). We named CRMs U1, U2 or D1, D2, and so on, according to their relative positions upstream or downstream from the TSS, respectively (see Figs 2 and 3 ). Notably, most head or trunk organizer genes examined, such as chordin , otx5 , wnt8a and not ( Fig. 3a,b ), possessed multiple CRMs occupied by Lim1, Otx2 and Gsc. Table 1 Overview of ChIP-seq peaks and CRMs. 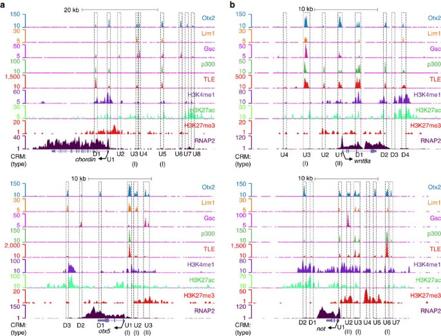Figure 3: Genome browser representations of ChIP-seq data around head and trunk organizer genes. (a) ChIP-seq data for head organizer genes,chordinandotx5. (b) ChIP-seq data for trunk organizer genes,wnt8aandnot. Genome browser representations were shown as inFig. 2a. Full size table Figure 3: Genome browser representations of ChIP-seq data around head and trunk organizer genes. ( a ) ChIP-seq data for head organizer genes, chordin and otx5 . ( b ) ChIP-seq data for trunk organizer genes, wnt8a and not . Genome browser representations were shown as in Fig. 2a . Full size image The X. tropicalis genome contains thousands of ‘potential CRMs’ (‘CRMs’ hereafter) bound by Otx2 (17,689), Lim1 (5,307) and Gsc (4,193), and most of them were co-occupied by p300 and TLE, suggesting that these CRMs function as enhancers, silencers or both in gastrula embryos ( Table 1 ). Although ChIP analyses were composites of binding data performed using whole embryos that comprise different cell types, it is reasonable to assume that most overlapping peaks indicate co-occupancy of Otx2, Lim1 and Gsc on the same CRM in the same cell, because these genes are predominantly coexpressed in the head organizer ( Fig. 1a ). We next asked whether Otx2-, Lim1- or Gsc-occupied CRMs have a tendency to co-occupy with p300 or TLE, which are designated as p300±TLE± (see four bottom rows in Table 1 ). Among 4,193 Gsc-binding CRMs, only 54 were p300+TLE− (1.3%), while 2,379 were p300−TLE+ (56.7%). By contrast, among 5,307 Lim1-binding CRMs, 1,224 were p300+TLE− (23.1%; much more than Gsc) and 765 were p300−TLE+ (14.4%; much less than Gsc). Otx2-binding CRMs showed 3,223 p300+TLE− (18.2%; similar to Lim1) and 6,793 p300−TLE+ (38.4%; between Lim1 and Gsc) among 17,689. This tendency for co-occupancy on CRMs between TFs and cofactors further confirmed the activator/repressor functions of Otx2, Lim1 and Gsc, as described above. Otx2 also colocalized frequently with Lim1 (4,937 CRMs), Gsc (3,401 CRMs) and with both (894 CRMs). However, colocalization of Lim1 and Gsc without Otx2 was much less common (12 CRMs). These observations imply that Otx2 cooperates with Lim1 and Gsc on distinct types of CRMs. TLE marks tissue-specific CRMs p300 occupancy can serve as a good predictor of tissue-specific enhancers by comparing different tissues isolated from mouse embryos [35] . However, because whole embryos were used for ChIP-seq analysis, it is conceivable that p300 binding is associated with both tissue-specific and ubiquitous enhancers, whereas TLE binding is associated with tissue-specific CRMs ( Fig. 4a ). We first tested whether p300 and TLE occupancies on CRMs are functionally associated with dorsal and ventral genes. We performed ChIP-qPCR for p300 and TLE using the dorsal and ventral halves of bisected gastrula embryos ( Fig. 4b ; see drawing) and calculated a D/V ratio of %recovery of each CRM (that is, %recovery in the dorsal half was divided by that in the ventral half; Fig. 4b ; see Supplementary Fig. 6 for details). As expected, p300 occupancies on 10 CRMs from dorsal genes exhibited significantly higher D/V ratios than those from ventral genes ( P =0.0035 in Fig. 4b ; left graph). Conversely, D/V ratios of TLE occupancies tended to be lower in the dorsal genes than in ventral genes ( Fig. 4b ; right graph). These data suggest that a majority of p300- and TLE-bound CRMs are functionally associated with tissue-specific genes. 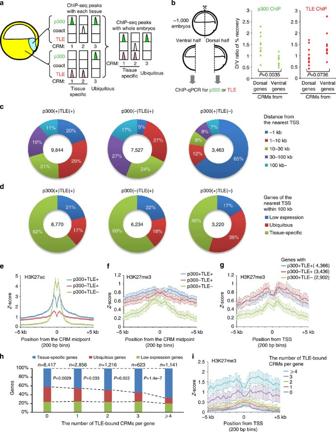Figure 4: Comprehensive analysis of tissue-specific gene regulation. (a) Schematic representation of ChIP-seq peaks for coactivators and corepressors with whole embryos. Virtual ChIP-seq peaks from the organizer (blue), the rest of the embryos (yellow) and whole embryos are shown. Tissue-specific CRMs 1 and 2 are occupied by either p300 or other coactivators (coact) in the organizer and mediate gene activation. When the same CRMs are occupied with TLE, silencing occurs somewhere in the non-organizer tissue. If ChIP-seq is performed using whole embryos, p300 binding identifies both ubiquitous enhancers (CRM 3) and tissue-specific enhancers (CRM 1). On the other hand, TLE binding is associated with only tissue-specific CRMs (CRMs 1 and 2). (b) ChIP-qPCR analysis for p300 and TLE using dorsal or ventral halves of gastrula embryos. Ten CRMs from both dorsal and ventral genes were examined. Ratios of %recovery of each CRM between dorsal and ventral halves (D/V) were plotted. Statistical significances of the difference between CRMs from dorsal and ventral genes were examined withχ2test. (c) Profiles of the distance between CRM and the nearest TSS. Pie charts show proportions of the distance for each group of CRMs as indicated. (d) Comparison of the tissue specificity of p300/TLE-bound CRMs. Pie charts show the proportions of CRMs assigned to genes in each group as indicated. (e,f) Epigenetic states around CRMs. AverageZ-scores of ChIP-seq signals of H3K27ac (e) or H3K27me3 (f) around the CRM midpoint were plotted with 95% confidence intervals as indicated as error bars. (g,i) Epigenetic states around TSSs. AverageZ-scores of ChIP-seq signals of H3K27me3 around TSSs assigned with CRMs within ±100 kb were plotted as inf. (h) Relationships between tissue specificity and the number of TLE-bound CRMs per gene. Bars represent percentages of three categories of genes from zero to more than three TLE-bound CRMs.Pvalues and statistical significances were calculated by theχ2test between two adjacent groups. Figure 4: Comprehensive analysis of tissue-specific gene regulation. ( a ) Schematic representation of ChIP-seq peaks for coactivators and corepressors with whole embryos. Virtual ChIP-seq peaks from the organizer (blue), the rest of the embryos (yellow) and whole embryos are shown. Tissue-specific CRMs 1 and 2 are occupied by either p300 or other coactivators (coact) in the organizer and mediate gene activation. When the same CRMs are occupied with TLE, silencing occurs somewhere in the non-organizer tissue. If ChIP-seq is performed using whole embryos, p300 binding identifies both ubiquitous enhancers (CRM 3) and tissue-specific enhancers (CRM 1). On the other hand, TLE binding is associated with only tissue-specific CRMs (CRMs 1 and 2). ( b ) ChIP-qPCR analysis for p300 and TLE using dorsal or ventral halves of gastrula embryos. Ten CRMs from both dorsal and ventral genes were examined. Ratios of %recovery of each CRM between dorsal and ventral halves (D/V) were plotted. Statistical significances of the difference between CRMs from dorsal and ventral genes were examined with χ 2 test. ( c ) Profiles of the distance between CRM and the nearest TSS. Pie charts show proportions of the distance for each group of CRMs as indicated. ( d ) Comparison of the tissue specificity of p300/TLE-bound CRMs. Pie charts show the proportions of CRMs assigned to genes in each group as indicated. ( e , f ) Epigenetic states around CRMs. Average Z -scores of ChIP-seq signals of H3K27ac ( e ) or H3K27me3 ( f ) around the CRM midpoint were plotted with 95% confidence intervals as indicated as error bars. ( g , i ) Epigenetic states around TSSs. Average Z -scores of ChIP-seq signals of H3K27me3 around TSSs assigned with CRMs within ±100 kb were plotted as in f . ( h ) Relationships between tissue specificity and the number of TLE-bound CRMs per gene. Bars represent percentages of three categories of genes from zero to more than three TLE-bound CRMs. P values and statistical significances were calculated by the χ 2 test between two adjacent groups. Full size image To further investigate relationships between CRMs and gene expression patterns, we next performed RNA-seq analysis with whole and dissected gastrula embryos (stage 10.5; Supplementary Fig. 7A–D ). Quality of dissection experiments was validated by reverse transcription qPCR (RT–qPCR) before sequencing ( Supplementary Fig. 7E–G ). RNA-seq short reads were mapped to the Xtev gene models [29] . We categorized them into three groups: (i) low or no expression (3,392 genes), (ii) tissue specific (6,562 genes) and (iii) ubiquitous (4,299 genes; see Supplementary Fig. 7A–D for definition). We then assigned previously identified CRMs to these genes. Because of the limitation of embryo dissection techniques, the ubiquitous group included relatively few tissue-specific genes, but the tissue-specific group did not include ubiquitous genes. Therefore, these categories were practical enough to use for the comprehensive analysis of genes as shown below. When we assigned each CRM to the nearest TSS, a large fraction of p300+TLE− CRMs (65%) were located within 1 kb of the nearest TSS ( Fig. 4c ). In contrast, only 20% of p300+TLE+ CRMs occurred within that range, and only 5% of p300−TLE+ CRMs ( Fig. 4c ). Furthermore, p300+TLE− CRMs within 1 kb of a TSS were strongly associated with ubiquitous genes ( P =9.01E−34, χ 2 test), whereas other p300+TLE− CRMs occurred almost randomly ( Supplementary Fig. 8 ). p300+TLE+ and p300−TLE+ CRMs (that is, TLE+ CRMs) were strongly associated with tissue-specific genes as long as CRMs were located within ±100 kb of their TSS ( P =1.05E−28 (p300+TLE+) and P =5.27E−26 (p300−TLE+) for CRMs within 30–100 kb of TSS, χ 2 test; see Supplementary Fig. 8 for details). These results suggest that p300+TLE− CRMs mainly regulate expression of ubiquitous genes close to the TSS and that p300+TLE+ and p300−TLE+ CRMs regulate expression of tissue-specific genes farther from the TSS ( Fig. 4d ). In other words, our data indicate that p300 occupancy alone does not predict tissue-specific CRMs and that TLE occupancy better predicts tissue-specific CRMs. Therefore, we assigned TLE-bound CRMs to the nearest TSS within a distance of 100 kb and focused on the relationship between TLE and function of tissue-specific CRMs. We next investigated epigenetic states around p300- or TLE-bound CRMs. As expected, p300-bound CRMs (p300+TLE+ and p300+TLE−) showed strong association with the active enhancer mark H3K27ac, whereas TLE showed an inverse association with it ( Fig. 4e ). Conversely, the repressive histone mark H3K27me3 was associated with TLE-bound CRMs (p300+TLE+ and p300−TLE+ CRMs) more strongly than with TLE-unbound CRMs (p300+TLE− CRMs; Fig. 4f ). At first inspection, it might appear problematic that Z -scores of H3K27me3 around TLE-bound CRMs were much smaller than those of H3K27ac around p300-bound CRMs ( Fig. 4e,f ). However, because the Z -score is defined as how many s.d. a datum is from the mean, these relatively low Z -scores of H3K27me3 were due to larger s.d. of H3K27me3 (8.55-fold of its mean), compared with those of H3K27ac (2.13-fold of its mean). These relatively high s.d. resulted from H3K27me3’s strongly biased distribution, as noted in previous reports [29] , [36] and exemplified by its high concentrations on ~5% of CRMs (see cluster 2 in Supplementary Fig. 9 ). Even so, a relatively greater enrichment of H3K27me3 was also observed around TSSs of genes with TLE-bound CRMs ( Fig. 4g ). This is in good agreement with a previous report that enrichment of H3K27me3 around TSSs is associated with spatially regulated genes [29] . We next examined the number of CRMs per gene within ±100 kb of the TSS and found that genes with more TLE-bound CRMs exhibit higher tissue specificity ( Fig. 4h ) and higher enrichment of H3K27me3 around TSS ( Fig. 4i ). These data suggest the possibility that TLE-bound CRMs function as silencers and that multiple TLE CRMs regulate tissue-specific genes. Combinatorial role of head organizer TFs in TLE-marked CRMs As mentioned above, we hypothesized that in the head organizer, in concert with Lim1 and Gsc, Otx2 activates and represses target genes, respectively. Because Otx2 target genes are supposedly tissue specific, we focused on Otx2/TLE-occupied CRMs to which Lim1 or Gsc are bound. Motif finding analyses were performed using Otx2/Lim1/TLE-occupied CRMs (3,066) and Otx2/Gsc/TLE-occupied CRMs (3,207), which only partially overlapped ( Fig. 5a ). We found that bicoid-binding motifs (TAATC(C/T)) [11] , [12] , [16] , [30] , which are bound by Otx2 and Gsc, and P3C motifs (bicoid/paired-type homo- or heterodimer-binding motifs (TAATCNNATTA)) [31] were enriched in Otx2/Gsc/TLE CRMs ( Fig. 5a ; Supplementary Fig. 10 ). However, bicoid-binding motifs were not enriched in Otx2/Lim1/TLE CRMs, despite the bound Otx2. In contrast, Lim1-binding motifs ((C/T)TAAT(G/T)(G/A)) [11] , [16] , [30] were enriched in Otx2/Lim1/TLE CRMs, but not in Otx2/Gsc/TLE CRMs ( Fig. 5a ; Supplementary Fig. 10 ). These data suggest that Lim1-, but not Otx2-binding motifs, are required for function of Otx2/Lim1/TLE CRMs, and that bicoid-binding motifs or P3C motifs are required for function of Otx2/Gsc/TLE CRMs. These observations were confirmed by two different algorithms, MEME-ChIP and Weeder ( Supplementary Fig. 10 ). We also noticed that the average number of Otx/Gsc-binding motifs in Otx2/Gsc/TLE CRMs is 1.24 motifs per CRM, which is significantly higher than the average in Otx2/TLE-occupied CRMs (0.70 motifs per CRM, P =2.5E−107, χ 2 test). This implies that CRMs with multiple Otx/Gsc-binding motifs are likely to function by binding both Otx2 and Gsc. Therefore, we further defined Otx2/Lim1/TLE CRMs containing Lim1-binding motifs as ‘type I’ CRMs (1,250 CRMs), and Otx2/Gsc/TLE CRMs containing multiple bicoid sites or P3C sites as ‘type II’ CRMs (1,039 CRMs; Fig. 5b ). We anticipate that genes with type I CRMs are activated in the head organizer, while those with type II CRMs are repressed ( Fig. 5b ). 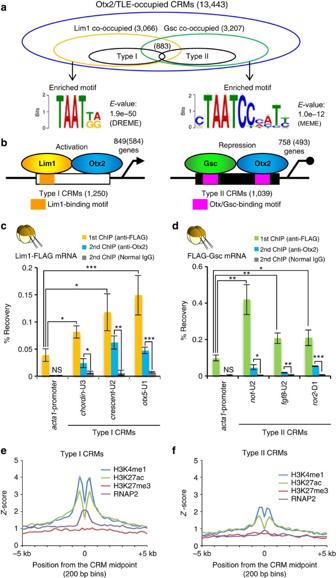Figure 5: Characterization of type I and type II CRMs. (a) Motif discovery analysis. Typical motifs enriched in Otx2/Lim1/TLE (3,066) and Otx2/Gsc/TLE (3,207) CRMs are shown withE-values. Algorithms used for motif discovery are indicated in parentheses (seeSupplementary Fig. 10for details). (b) Definition of type I and type II CRMs. The number of genes assigned with type I or type II CRMs alone is shown in parentheses. (c,d) Sequential ChIP assay. Embryos injected with mRNA-encoding FLAG-tagged Lim1 (c) or Gsc (d) were used. qPCR data for first ChIP (anti-FLAG) shows significant enrichment of type I or type II CRMs bound by FLAG-tagged Lim1 or Gsc, respectively, compared with the negative control region (acta1-promoter). qPCR data for second ChIP shows significant enrichment of each CRM by anti-Otx2 compared with the negative control (normal IgG). Bar graphs show %recovery of DNA±s.d. *P<0.05; **P<0.01; ***P<0.001 (t-test, two tailed). (e,f) Epigenetic analysis. Enhancer histone marks, H3K4me1 and H3K27ac, were enriched around type I CRMs. RNA polymerase II (RNAP2) was also enriched at the midpoint of type I CRMs (e). However, these marks were relatively poor around type II CRMs (f). Figure 5: Characterization of type I and type II CRMs. ( a ) Motif discovery analysis. Typical motifs enriched in Otx2/Lim1/TLE (3,066) and Otx2/Gsc/TLE (3,207) CRMs are shown with E -values. Algorithms used for motif discovery are indicated in parentheses (see Supplementary Fig. 10 for details). ( b ) Definition of type I and type II CRMs. The number of genes assigned with type I or type II CRMs alone is shown in parentheses. ( c , d ) Sequential ChIP assay. Embryos injected with mRNA-encoding FLAG-tagged Lim1 ( c ) or Gsc ( d ) were used. qPCR data for first ChIP (anti-FLAG) shows significant enrichment of type I or type II CRMs bound by FLAG-tagged Lim1 or Gsc, respectively, compared with the negative control region ( acta1 -promoter). qPCR data for second ChIP shows significant enrichment of each CRM by anti-Otx2 compared with the negative control (normal IgG). Bar graphs show %recovery of DNA±s.d. * P <0.05; ** P <0.01; *** P <0.001 ( t -test, two tailed). ( e , f ) Epigenetic analysis. Enhancer histone marks, H3K4me1 and H3K27ac, were enriched around type I CRMs. RNA polymerase II (RNAP2) was also enriched at the midpoint of type I CRMs ( e ). However, these marks were relatively poor around type II CRMs ( f ). Full size image To ensure that Otx2 interacts with Lim1 or Gsc on type I or type II CRMs, respectively, we performed sequential ChIP assays ( Fig. 5c,d ). For this assay, we analysed interactions between endogenous Otx2 proteins and exogenous Lim1 or Gsc, because %recoveries of target CRMs by ChIP-qPCR using Lim1 and Gsc antibodies were fairly low compared with those using Otx2 antibodies (see Supplementary Fig. 4A–C ). mRNA for FLAG-tagged Lim1 or Gsc was injected into the dorsal equatorial region of four-cell X. laevis embryos. Chromatin from gastrula embryos was first immunoprecipitated with anti-FLAG antibody, followed by a second ChIP with either anti-Otx2 antibody or pre-immune rabbit IgG (negative control). qPCR for selected type I or II CRMs, the sequences of which, including binding motifs, are largely conserved in X. tropicalis and X. laevis , demonstrated that FLAG-tagged Lim1 was associated with endogenous Otx2 protein on type I CRMs and that FLAG-tagged Gsc was associated with Otx2 on type II CRMs ( Fig. 5c,d ). These results suggest that Lim1 and Gsc can make a complex with Otx2 on CRMs, further supporting our combinatorial regulatory model ( Fig. 5b ). Consistent with our expectations, epigenetic analysis of CRMs revealed that type I CRMs, but not type II CRMs, are closely associated with H3K4me1, H3K27ac and RNAP2 ( Fig. 5e,f ), suggesting that type I CRMs tend to function as enhancers. However, it should be noted that our definition of types I and II is not mutually exclusive. Some CRMs (141) were categorized as both types I and II, for example, gsc -U1. This kind of CRM might be activated by Lim1 and repressed by Gsc, as has been shown for gsc -U1 (ref. 11 ) (see Fig. 2a ). Reporter analysis for type I and type II CRMs We next examined responsiveness of individual type I and type II CRMs towards Otx2, Lim1 and Gsc, using reporter assays in which a reporter gene and the ‘head organizer cocktail’ (see Fig. 1c ) were coinjected in the animal pole region. The head organizer cocktail activated 15 of 16 luciferase reporter genes harbouring type I CRMs derived from 9 head organizer genes and 3 trunk genes ( Fig. 6a ). To examine repressive activity of type II CRMs, we used SV40 late promoter for raising basal transcriptional activity (see Methods for more details of reporter constructs). In this assay, the same cocktail repressed the activity of reporter genes harbouring eight of nine type II CRMs derived from six trunk genes and three head organizer genes. These data suggest that type I and type II CRMs function as enhancers and silencers, respectively, in the head organizer, irrespective of their component genes, justifying our two-CRM classification. We next examined the dependency of responsiveness on binding motifs. Reporter constructs with mutated Lim1- or Otx2/Gsc-binding motifs in CRMs exhibited significantly reduced responsiveness ( Fig. 6b ). Thus, reporter analysis of individual CRMs strongly supported the classification of type I and type II CRMs ( Fig. 5b ). 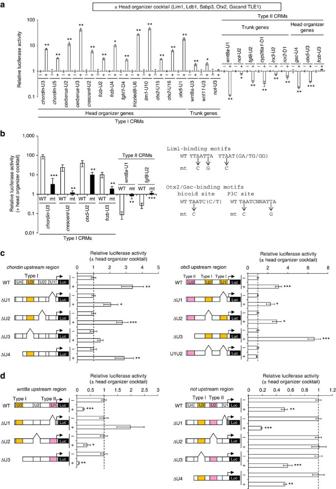Figure 6: Enhancer or silencer activities of type I and type II CRMs inX. laevisembryos. (a) Luciferase reporter assay for type I and type II CRMs isolated from various genes. (b) Mutation analysis for binding motifs. Responses to the head organizer cocktail were compared between wild type (WT) and mutant (mt) CRMs as indicated. Mutated sequences of binding motifs are shown on the right. (c,d) Luciferase reporter assay for 4–9 kb upstream regions of head organizer genes (c) and trunk genes (d). Deletion constructs for each CRM were examined as indicated. Type I and type II CRMs are shown with orange and magenta boxes, respectively. For thenotΔU1 construct, the inserted SV40 promoter is indicated as a grey box (see Methods for details). Bars represent the mean±s.e.m. of luciferase activities relative to the mean value obtained from a reporter without the head organizer cocktail. These results show that the head organizer cocktail activates and represses target genes through type I and type II CRMs, respectively, in a binding motif-dependent manner. Basically, the results from an experiment are shown for each reporter construct, except fornot-U2 inaandchordinupstream region constructs inc, in which the results of two independent experiments were combined. *P<0.05; **P<0.01; ***P<0.01 (t-test, two tailed). Figure 6: Enhancer or silencer activities of type I and type II CRMs in X. laevis embryos. ( a ) Luciferase reporter assay for type I and type II CRMs isolated from various genes. ( b ) Mutation analysis for binding motifs. Responses to the head organizer cocktail were compared between wild type (WT) and mutant (mt) CRMs as indicated. Mutated sequences of binding motifs are shown on the right. ( c , d ) Luciferase reporter assay for 4–9 kb upstream regions of head organizer genes ( c ) and trunk genes ( d ). Deletion constructs for each CRM were examined as indicated. Type I and type II CRMs are shown with orange and magenta boxes, respectively. For the not ΔU1 construct, the inserted SV40 promoter is indicated as a grey box (see Methods for details). Bars represent the mean±s.e.m. of luciferase activities relative to the mean value obtained from a reporter without the head organizer cocktail. These results show that the head organizer cocktail activates and represses target genes through type I and type II CRMs, respectively, in a binding motif-dependent manner. Basically, the results from an experiment are shown for each reporter construct, except for not -U2 in a and chordin upstream region constructs in c , in which the results of two independent experiments were combined. * P <0.05; ** P <0.01; *** P <0.01 ( t -test, two tailed). Full size image As mentioned above, head and trunk organizer genes have multiple CRMs, which may be type I, type II or both ( Figs 2a and 3 ). To examine whether type I and type II CRMs participate in regulation of target genes, and to determine how type I and type II CRMs interact with each other, when coexisting in the same genes, we prepared reporter constructs connected with 4–9 kb upstream regions for chordin , otx5 , wnt8a, and not , which possess 3–4 TLE-bound CRMs ( Fig. 6c,d ). Results of reporter analyses with a series of deletion constructs showed that type I CRMs in chordin and otx5 reporter constructs are necessary for the head organizer cocktail to activate the luciferase reporter gene ( Fig. 6c ). Furthermore, in otx5 , two type I CRMs, U1 and U2, functioned redundantly, and the type II CRM, U3, functioned as a silencer. Because Otx5 has basically the same activity as Otx2, U3 is likely to play a role in autorepression, as has been shown for gsc [11] , [32] . Concerning trunk organizer genes, type II CRMs in wnt8a (U1) and not (U2) reporter constructs are necessary for the head organizer cocktail to repress the luciferase reporter gene ( Fig. 6d ). Deletion of type I wnt8a -U3 enhanced repression by the head organizer cocktail, whereas deletion of type I not -U3 did not, consistent with the high activity of wnt8a -U3 and near inactivity of not -U3 in reporter assays using a single copy of type I CRMs (see Fig. 6a ). These data suggest that type I or type II CRM independently activates or represses target genes, respectively, in the head organizer context. Type I and type II CRM function in the head organizer To test whether type I and type II of CRMs are correlated with gene expression in the embryo, we examined expression profiles in lim1/otx2/otx5 morphants and gsc morphants using RNA-seq analysis. We categorized all expressed genes into up- or downregulated genes in morphants compared with two controls, uninjected embryos and standard control MO-injected embryos (control morphants). Among these categories, Otx2/TLE, Lim1/TLE and type I CRMs were enriched around downregulated genes in lim1/otx2/otx5 morphants ( Supplementary Fig. 11A ). Similarly, Gsc and Gsc/TLE CRMs were enriched around both up- and downregulated genes in gsc morphants, and type II CRMs were enriched around those upregulated genes ( Supplementary Fig. 11B ). These results suggested that Otx2, Lim1 and Gsc CRMs including type I and type II CRMs were functionally correlated with proximal gene expression. We further examined type I CRMs’ functions in the head organizer. Utilizing RNA-seq results of dissected head organizer regions ( Supplementary Fig. 7B ), we identified 87 genes that were enriched greater than fivefold in the head organizer region compared with other embryonic regions. We called them ‘head organizer genes,’ because the list included all 23 known head organizer genes and 5 dorsal endodermal genes, but did not include trunk organizer, pan-mesodermal, pan-endodermal, intermediate mesodermal or neural ectodermal genes ( Supplementary Data 1 ). Therefore, the list appears to represent a complete compilation of head organizer genes. RNA-seq analysis using lim1/otx2/otx5 morphants showed that expression levels of the head organizer genes possessing type I CRMs were significantly reduced in lim1/otx2/otx5 morphants ( Fig. 7a ) compared with control morphants ( P =0.0068), and also tended to be lowered than those of genes lacking type I CRMs ( P =0.054). This result suggests that head organizer genes possessing type I CRMs are positively regulated by Lim1 and Otx2 in vivo , possibly through type I CRMs. 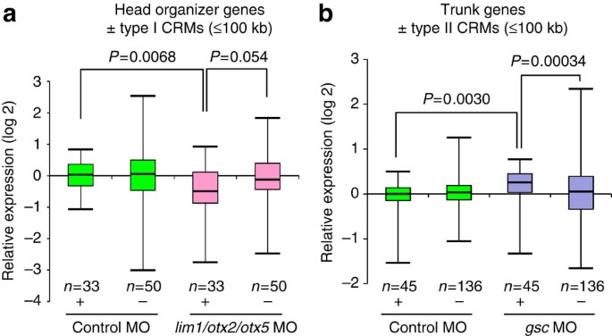Figure 7: Requirement of type I and type II CRMs for gene activation and repression in the head organizer. (a) Head organizer genes with and without type I CRMs. Eighty-three of the 87 comprehensively identified head organizer genes were used (listed inSupplementary Data 1). Gene expression levels analysed by RNA-seq showing log2 ratios of injected embryos versus uninjected controls. Expression levels in control orlim1/otx2/otx5morphants were analysed at the mid-gastrula stage (stage 11.5). (b) Trunk genes with and without type II CRMs. The 181 comprehensively identified trunk genes were used (listed inSupplementary Data 2). Expression levels in control orgscmorphants were analysed at the mid-gastrula stage (stage 11). Expression levels were compared byχ2test andPvalues are shown. The results indicate that Lim1/Otx2/Otx5 upregulates head organizer genes with type I CRMs and that Gsc downregulates trunk genes with type II CRMs. Relative expression levels were displayed as box-and-whisker plots; boxes represent 25–75%, the line with the box indicates the median and whiskers represent from minimum to maximum, respectively. Figure 7: Requirement of type I and type II CRMs for gene activation and repression in the head organizer. ( a ) Head organizer genes with and without type I CRMs. Eighty-three of the 87 comprehensively identified head organizer genes were used (listed in Supplementary Data 1 ). Gene expression levels analysed by RNA-seq showing log2 ratios of injected embryos versus uninjected controls. Expression levels in control or lim1/otx2/otx5 morphants were analysed at the mid-gastrula stage (stage 11.5). ( b ) Trunk genes with and without type II CRMs. The 181 comprehensively identified trunk genes were used (listed in Supplementary Data 2 ). Expression levels in control or gsc morphants were analysed at the mid-gastrula stage (stage 11). Expression levels were compared by χ 2 test and P values are shown. The results indicate that Lim1/Otx2/Otx5 upregulates head organizer genes with type I CRMs and that Gsc downregulates trunk genes with type II CRMs. Relative expression levels were displayed as box-and-whisker plots; boxes represent 25–75%, the line with the box indicates the median and whiskers represent from minimum to maximum, respectively. Full size image Finally, we examined type II CRMs’ functions in trunk genes, which are supposed to be repressed in the head organizer. We identified 181 ‘trunk genes’ ( Supplementary Data 2 ) that were enriched greater than threefold in the marginal zone ( Supplementary Fig. 7C ) and were not included among the 87 head organizer genes. Trunk genes include 68 known posterior mesodermal genes such as wnt8a , vegt and brachyury . RNA-seq results showed that trunk genes possessing type II CRMs were significantly upregulated in gsc morphants ( Fig. 7b ), compared with control morphants ( P =0.0030) and with trunk genes lacking type II CRMs ( P =0.00034). This result supports the idea that trunk genes possessing type II CRMs are negatively regulated by Gsc, possibly through type II CRMs. We have shown that the corepressor TLE/Groucho identifies tissue-specific CRMs in the embryo. This is paradoxical, but it makes sense because activating a certain gene in a specific region results in its repression elsewhere. Similarly, it was recently reported that most regions bound by PRC2 subunits Ezh2 and Jarid2 had the enhancer histone mark H3K4me1 in Xenopus embryos [36] . Furthermore, we have shown the importance of multiple TLE-marked CRMs for tissue-specific expression. This finding is reminiscent of a recently reported ‘super-enhancer’ in which clusters of enhancers are occupied by the master TFs and the mediator coactivator complex to regulate ‘cell identity genes’ [37] . If up- and downregulation are ‘two sides of the same coin,’ repression of cell identity genes requires TLE to bind to each CRM in the super-enhancer. Thus, TLE is a very useful marker for tissue-specific CRMs in comprehensive genome-wide analysis. Utilizing TLE as a tissue-specific CRM marker, we were able to identify type I and type II CRMs ( Fig. 5a,b ) that activate or repress a large battery of genes, including head organizer and trunk genes ( Figs 6 and 7 ). We estimated the number of Otx2 target genes that have type I, type II or both, to be 584, 493 or 265, respectively, in the Xenopus gastrula ( Fig. 5b ). On the basis of these data, we propose a regulatory principle, in which the selector, Otx2, acts as a ‘molecular landmark’ of the head organizer by positively or negatively regulating hundreds of target genes in cooperation with Lim1 or Gsc, through type I or type II CRMs, respectively ( Supplementary Fig. 1B ). This regulatory principle may also apply to other bilaterians because of evolutionary conservation of Otx/Otd in head formation [2] , but activators and repressors as partner TFs of Otx can be different from organism to organism, depending on different developmental processes for diverse bilaterian head structures. ChIP-chip analyses of a Drosophila Hox protein, Ubx, using the haltere disc have identified Ubx peaks near 1,147–3,400 genes, which were either activated or repressed by Ubx [38] , [39] . In addition, whole-genome ChIP-chip analyses of Dorsal, Twist and Snail in Drosophila have also shown similar results [40] , [41] , in which these TFs appeared to exert positive/negative regulation on hundreds to thousands of target genes for dorsoventral patterning, anteroposterior patterning and mesoderm differentiation. Our ChIP-seq analyses for Otx2, Lim1 and Gsc in early vertebrate embryos are consistent with work in Drosophila . Moreover, our data highlight a general gene regulatory principle that, although the selector TF itself appears to have dual functions, selector TFs may only mark target genes to be regulated. Then, partner TFs may activate or repress selector-marked target genes, depending on the biological context. Reporter assays for type I and type II CRMs showed that Lim1- and Otx2/Gsc-binding motifs in CRMs are important to regulate genes ( Fig. 6b ). Curiously, even though Otx2 binds to type I CRMs, 56.4% of type I CRMs do not contain typical Otx2-binding motifs, suggesting that Otx2 may bind to atypical motifs or function as a coactivator for Lim1 without directly binding to DNA. This possibility is supported by sequential ChIP assays, which confirmed that Otx2 complexes with Lim1 on three type I CRMs that do not contain typical Otx2-binding motifs ( Fig. 5c ). Because some homeodomain proteins, such as Gsc, Pbx1 and Meis1 [42] , [43] , can function without direct DNA binding, Otx2 may also function similarly. By contrast, for repressing target genes through type II CRMs, Otx2 probably needs to bind to bicoid sites. The switching mechanism between activator and repressor activities of Otx2 could be uncovered by deeper ChIP-seq and RNA-seq analyses in future. Animals Adult males and females of X. laevis were purchased from Sato Breeder (Japan), and maintained in our frog facility. Adult males and females of X. tropicalis were obtained from the National Bioresource Project and bred in our frog facility. All experiments with X. tropicalis and X. laevis were approved by the Animal Care and Use Committees in the University of Tokyo and Okinawa Institute of Science and Technology Graduate University. Microinjection experiments in Xenopus embryos X. tropicalis ’ and X. laevis ’ fertilized eggs were dejellied and injected with MOs and mRNAs. For mRNA synthesis, coding sequences of Xenopus genes used in this study were cloned into the pCSf107mT vector, which contains SP6/T7 terminator sequences [44] . Capped mRNA was synthesized using the mMESSAGE mMACHINE SP6 kit (Ambion). For X. tropicalis embryos, MOs were injected at the animal pole of both blastomeres at the two-cell stage, because MOs diffuse throughout the blastomere to knockdown target genes in the entire embryo. Phenotypes of morphants were scored at the tailbud stage. Some of them were subjected to sagittal sections stained with haematoxylin and eosin (Biopathology Institute, Oita, Japan). MOs were purchased from Gene Tools. MO sequences are as follows (antisense start codons are underlined): standard control MO, 5′-CCTCTTACCTCAGTTACAATTTATA-3′; lim1 MO, 5′-TTTCGCATCCAGCACAGTGAAC CAT -3′; otx2 MO, 5′-GGTTGCTTGAGATAAGACAT CAT GC-3′; otx5 MO, 5′-AATGTAGGACAT CAT TTCAGTGGCC-3′; gsc MO, 5′-GCTGAACATGCCAGAAGG CAT CACC-3′ (ref. 24 ). For RNA-seq with loss-of-function experiments, a cocktail of lim1, otx2, otx5 MOs (0.75 pmol per embryo each), standard control MO (2.25 pmol per embryo) or gsc MO (2.25 pmol per embryo) was injected. For secondary head formation, 25 pg of lim1 , ldb1 and ssbp3 , 20 pg of otx2 and tle1 or 10 pg of gsc mRNAs were injected in various combinations into single blastomeres in the ventral equatorial region of four-cell X. laevis embryos. For animal cap assays using X. laevis embryos, mRNAs for lim1 , ldb1 , ssbp3 , otx2 , gsc and tle1 (25, 25, 25, 20, 10 and 20 pg per embryo, respectively) or gfp (150 pg per embryo) were injected into the animal pole region of both blastomeres at the two-cell stage. Animal caps were dissected from blastulae (stages 8.5–9) and collected at the stage equivalent to the gastrula or neurula stage for analysing gene expression as described [45] . Total RNA was extracted using ISOGEN (Wako, Japan) from 10 caps or three embryos and used for RT–qPCR. Whole-mount in situ hybridization Whole-mount in situ hybridization was carried out as described [46] . Briefly, X. tropicalis embryos were fixed with MOPS/EGTA/magnesium sulfate/formaldehyde buffer (MEMFA; 100 mM MOPS, pH7.4, 2 mM EGTA, 1 mM MgSO 4 , and 3.7% formaldehyde) for 1.5–3 h at room temperature and dehydrated with ethanol. For hemisections, rehydrated embryos were embedded in 2% low-melting point agarose with 0.3 M sucrose in 1 × phosphate-buffered saline (PBS). Agarose-mounted embryos were bisected and refixed with MEMFA for 30 min at room temperature as described [16] . Proteinase K treatment was carried out at 1.25 μg ml −1 for 30 min (whole embryos) or at 0.625 μg ml −1 for 20 min (hemisections). Embryos or hemisections were hybridized with digoxigenin-labelled antisense RNA probes, which were transcribed from linearized plasmids containing full coding sequences of X. tropicalis genes, except for gsc whose sequence is obtained from X. laevis (92% identical with that of X. tropicalis ). After treatment with alkaline phosphatase-conjugated anti-DIG antibody (Roche; 1/2,000 diluted), chromogenic reaction was performed with BM Purple (Roche). Stained embryos were bleached and observed under the stereomicroscope (Leica M205 FA). Whole-mount immunostaining Whole-mount immunostaining were performed as described [45] , [47] . Briefly, X. laevis embryos were fixed with MEMFA for 1.5–3 h at room temperature and dehydrated with methanol. Rehydrated embryos were blocked in 1 × Tris-buffered saline (TBS) containing BSA/TritonX-100/Serum (TBTS; 25 mM Tris–Cl, pH 7.4, 137 mM NaCl, 2.7 mM KCl, 0.2% bovine serum albumin, 0.1% Triton X-100 and 10% lamb serum), and reacted with the primary antibody overnight at 4 °C, followed by the secondary antibody reaction. For notochord staining, MZ15 (a gift from Dr F. Watt) was used as the primary antibody (1/500 diluted), alkaline phosphatase-conjugated anti mouse IgG was used as the secondary antibody (Promega, 1/500 diluted) and BM Purple was used for chromogenic reaction. For somites’ staining, 12/101 (obtained from the Developmental Studies Hybridoma Bank, the University of Iowa) was used as the primary antibody (1/100 diluted), horseradish peroxidase-conjugated anti mouse IgG was used as the secondary antibody (Promega, 1/500 diluted) and 3,3′-diaminobenzidine was used for chromogenic reaction. Bleached embryos were cleared with benzyl benzoate/benzyl alcohol (2:1) and observed under the stereomicroscope (Leica M205 FA). qPCR qPCR was performed using SYBR Green. Primer sequences for ChIP-qPCR and RT-qPCR are described in Supplementary Tables 3 and 4 , respectively. For ChIP-qPCR using X. laevis embryos, PCR amplicons and primer sets were determined according to sequence conservation in X. tropicalis and X. laevis , using genome data on Xenbase ( http://www.xenbase.org/common/ ). For RT-qPCR using X. laevis and X. tropicalis , relative expression levels of genes were calculated after normalization with the expression level of ef1 α. Antibodies for ChIP analysis Anti-Lim1 and anti-Otx2 antibodies (1 mg ml −1 and 0.4 mg mg −1 , respectively) were raised and affinity purified [16] . Anti-p300 and anti-pan-TLE antibodies were purchased from Santa Cruz (sc-585 and sc-13373, 2 mg ml −1 ), and anti-H3K4me1 and anti-H3K27ac antibodies were purchased from Abcam (ab8895 and ab4729, 1 mg ml −1 ). Specificity of anti-Otx2 antibody was validated by immunoprecipitation and western blotting with embryos injected with otx2 mRNA at 500 pg per embryo ( Supplementary Fig. 4F ). Gsc antibody (0.01 mg ml −1 ) was raised against the amino terminus (167 aa) of the protein and affinity purified. Specificity of anti-Gsc antibody was validated by western blotting with embryos injected with FLAG- gsc mRNA at 250 pg per embryo ( Supplementary Fig. 4G ). The X. tropicalis p300 carboxy-terminal sequence is 85% identical to the epitope derived from human p300 (17/20 aa), which includes a 10-aa match at the C terminus. The epitope of anti-pan-TLE antibody is 100%, 89.4% and 100% identical to the C terminus of X. tropicalis TLE1, TLE2/3 and TLE4, respectively. ChIP-seq analysis Chromatin extraction from X. tropicalis embryos was performed as previously described [16] , [48] , with slight modifications. Briefly, X. tropicalis gastrula embryos were fixed at 25 °C with 1% formaldehyde in 1 × PBS for 30 min, further incubated for 10 min after addition of 1/9 volume of 1.25 M glycine and rinsed with 10 mM Tris–HCl (pH 7.5) or 1 × PBS twice. Fixed embryos were homogenized with a Dounce homogenizer in 2.2 M sucrose, 10 mM Tris–HCl (pH 7.5), 3 mM CaCl 2 , 0.5% Triton X-100 and proteinase inhibitor cocktail (50 μg ml −1 aprotinin, 20 μg ml −1 pepstatin A, 40 μg ml −1 leupeptin and 1 mM phenylmethylsulphonyl fluoride). Homogenates were centrifuged at 4 °C for 3 h at 8,000 g . Precipitated nuclei were rinsed twice with 250 mM sucrose, 10 mM Tris-HCl (pH 7.5), 3 mM CaCl 2 and proteinase inhibitors. Nuclei were sonicated in lysis buffer 3 (Agilent Mammalian ChIP-on-chip Protocol; 10 mM Tris–HCl, pH 8.0, 100 mM NaCl, 1 mM EDTA, 0.5 mM EGTA, 0.1% Na-deoxycholate and 0.5% N -lauroylsarcosine) with the protease inhibitor cocktail, shearing chromatin into 100–200 bp fragments. Sheared chromatin from 2,000–3,000 X. tropicalis gastrula embryos (~stage 10.5) in lysis buffer 3 containing 1% Triton X-100 was immunoprecipitated with 30 μg of antibodies and 300 μl of Dynabeads protein A (Invitrogen), except for anti-Gsc (1 μg of antibodies and 100 μl of Dynabeads protein A), according to the Agilent protocol. ChIP efficiency was greater than or equal to threefold higher than that for a control genomic region, as determined by qPCR ( Supplementary Fig. 4A–E ). For ChIP-qPCR assay using bisected embryos, ~1,000 fixed early gastrula embryos were bisected into dorsal and ventral halves. Sheared chromatin from dorsal or ventral halves was immunoprecipitated with 10 μg of p300 or TLE antibodies. ChIP DNA and input control DNA were sequenced using Illumina GAIIx as previously described [49] , [50] . Sequence tags (36 bases) were mapped to the X. tropicalis genome, Joint Genome Institute, assembly version 4.1, using ELAND (Illumina). Uniquely mapped sequences allowing up to two mismatches were extracted and computationally extended to the average DNA fragment size used for sequencing (120 bases). Using seqMINER [51] , the mapping data were subjected to k -means clustering and visualized as heatmaps. A genome representation was generated using the UCSC genome browser. Wiggled files of ChIP-seq data for genome browser representation are available as Supplementary Data 3–9 . To detect binding peaks, enrichment against an input control (IP/WCE) was calculated using tag concentrations per genome position [49] . For calculations of Z -scores and Pearson correlation coefficient, the average enrichment data of each TF in 200 bp bins were used. The definition of ChIP-seq peaks was more than five- (Lim1 and Gsc) or tenfold (Otx2, p300 and TLE) enrichment (over control) and more than 120 bases in length (see Supplementary Table 1 ). Because of the low efficiency of ChIP experiments with anti-Lim1 and anti-Gsc antibodies (see Supplementary Fig. 4A,C ), the peak detection threshold was set at greater than fivefold for Lim1 and Gsc (false discovery rate<0.01; see Supplementary Table 1 ). Our peak detection algorithm was compared with MACS ( http://liulab.dfci.harvard.edu/MACS/ ; Supplementary Table 2 ). Peaks that shared >120 bases were considered overlapping. Consecutively overlapping peaks were combined as a single CRM spanning the overlapping peaks. Genomic positions of CRMs and ChIP-seq peaks are available as Supplementary Data 10 . The number of Lim1- or bicoid/P3C-binding motifs was counted for Lim1 or Otx2 peaks in CRMs. If the TSS occurred within the CRM, the distance was considered zero. Motifs enriched in ChIP-seq peaks and CRMs were analysed by MEME-ChIP [52] and Weeder [53] with settings to consider both strands, to find one or more motifs in some sequences and to find the motif width from 6 to 15 for the MEME algorithm. RNA-seq analysis Total RNA was extracted using ISOGEN (Wako) from ~10 X. tropicalis embryos that had been injected with MO, or from a set of dissected tissues from early gastrula embryos (see Supplementary Fig. 7B–D ). RNA-seq was performed using Illumina GAIIx as previously described [49] , [54] . Sequence tags (36 bp) were mapped to the 14,253 Xtev gene models [29] and two JGI gene models, e_gw1.925.59.1 and gw1.925.54.1 ( siamois2 / twin and siamois3 , respectively) using ELAND. Uniquely mapped sequences without any mismatches were used to calculate RPKM (reads per kilobase of exon per million mapped reads) for each gene model. RPKM values were used for comparisons of expression levels of each gene. Sequential ChIP assay For sequential ChIP assays, we fixed X. laevis gastrula embryos as described above and extracted chromatin as follows. Fixed embryos were homogenized with a Dounce homogenizer in lysis buffer 1 (Agilent Protocol; 50 mM Hepes-KOH, pH 7.5, 140 mM NaCl, 1 mM EDTA, 10% glycerol, 0.5% Igepal and 0.25% Triton X-100) with proteinase inhibitor cocktail (complete, Roche), and rocked at 4 °C for 10 min. Homogenates were centrifuged at 4 °C for 5 min at 1,500 g . Precipitated nuclei were resuspended in lysis buffer 3 with proteinase inhibitor cocktail and sonicated. Sheared chromatin was obtained from 300 X. laevis gastrula embryos (~stage 10.5) injected with 250 pg of mRNA encoding C-terminally FLAG-tagged Lim1 or N-terminally FLAG-tagged Gsc into two blastomeres of the dorsal equatorial region at the four-cell stage. Chromatin was first immunoprecipitated with 100 μl of anti-FLAG M2 magnetic beads (Sigma, M8823) as described above, except that chromatin was eluted in 300 μl of Tris/EDTA buffer (TE; 10 mM Tris-Cl, 1 mM EDTA, pH 8.0) with 30 mM dithiothreitol, 500 mM NaCl and 0.1% SDS at 37 °C for 30 min as previously described [55] . Eluted chromatin (100 μl) was kept as a first ChIP sample. The other 100 μl of eluted chromatin was diluted tenfold with lysis buffer 3 (Agilent Protocol) containing 1% Triton X-100 and subjected to a second immunoprecipitation with 10 μg of anti-Otx2 antibody or normal rabbit IgG (CST, #2729). Isolated DNA was purified and examined by qPCR. Reporter constructs and luciferase assay Luciferase reporter constructs for type I CRMs were made by inserting a genomic fragment into the pGL4.23 vector (Promega), which has an artificial, minimal promoter. To examine type II CRMs for gene repression, the minimal promoter was replaced with the SV40 late promoter. Because wnt8a -U1 includes original promoter sequences, the wnt8a -U1 genomic fragment was inserted into the pGL4.23 vector. To make reporter constructs shown in Fig. 6c,d , 5′ upstream regions from start codons of genes were connected to the start codon of the luciferase reporter gene. To make ΔU1 constructs ( Fig. 6d ), the previously reported minimal promoter sequence [15] was left for the wnt8a construct, whereas SV40 promoter was inserted for the not construct because not -U1 overlaps the start codon and its minimal promoter sequence was unclear. Luciferase assays using X. laevis embryos were performed as previously described [12] , [45] . Reporter plasmid DNA (50 pg per embryo) with mRNAs for lim1 , ldb1 , ssbp3 , otx2 , gsc and tle1 (25, 25, 25, 20, 10 and 20 pg per embryo, respectively) were injected together into the animal pole region of both blastomeres at the two-cell stage. Luciferase activity was analysed at the gastrula stage (stage 10.5–11). The mean and standard error were calculated by assaying five pools of three embryos for each injection sample. Accession Codes : Short-read sequence data for ChIP-seq and RNA-seq analyses have been deposited in the DDBJ Sequence Read Archive (DRA) under accession codes DRA000505, DRA000506 and DRA000507 (ChIP-seq for p300, TLE and input control); DRA000508, DRA000509 and DRA000510 (ChIP-seq for Otx2, Lim1 and input control); DRA000573, DRA000574 and DRA000575 (ChIP-seq for H3K4me1, H3K27ac and input control), DRA000576 and DRA000577 (ChIP-seq for Gsc and input control); DRA000514 and DRA000515 (RNA-seq for dissected head organizer regions and remaining regions); DRA000516, DRA000517 and DRA000518 (RNA-seq for lim1/otx2/otx5 knockdown embryos and control embryos); DRA000642 and DRA000732 (RNA-seq for dissected marginal zone and remaining regions); DRA000645, DRA000648 and DRA000649 (RNA-seq for dissected dorsal regions, ventral regions and whole embryos); and DRA001093, DRA001094 and DRA001095 (RNA-seq for gsc knockdown embryos and control embryos). How to cite this article: Yasuoka, Y. et al. Occupancy of tissue-specific cis -regulatory modules by Otx2 and TLE/Groucho for embryonic head specification. Nat. Commun. 5:4322 doi: 10.1038/ncomms5322 (2014).